Documentation and localization of force-mediated filamin A domain perturbations in moving cells Endogenously and externally generated mechanical forces influence diverse cellular activities, a phenomenon defined as mechanotransduction. Deformation of protein domains by application of stress, previously documented to alter macromolecular interactions in vitro , could mediate these effects. We engineered a photon-emitting system responsive to unfolding of two repeat domains of the actin filament (F-actin) crosslinker protein filamin A (FLNA) that binds multiple partners involved in cell signalling reactions and validated the system using F-actin networks subjected to myosin-based contraction. Expressed in cultured cells, the sensor-containing FLNA construct reproducibly reported FLNA domain unfolding strikingly localized to dynamic, actively protruding, leading cell edges. The unfolding signal depends upon coherence of F-actin-FLNA networks and is enhanced by stimulating cell contractility. The results establish protein domain distortion as a bona fide mechanism for mechanotransduction in vivo . The actin cytoskeleton provides shape and mechanical stability to cells, and bidirectional signals between the cytoskeleton and membrane receptors and adhesion proteins regulate cell shape and movement. While chemical signals downstream of receptor ligation, such as ATP hydrolysis and phosphorylation can mediate cytoskeletal rearrangements, force-dependent conformational changes of load-bearing molecules can generate mechanotransduction, where mechanical forces are converted to biochemical signals [1] , [2] , [3] , [4] , [5] , [6] . However, little information is available concerning the spatio–temporal regulation of such molecules in cells primarily due to a limitation of reagents capable of detecting force-induced conformational change in situ [6] . Obtaining such information is potentially important, because mechanical strain has medical consequences such as pathological vascular and cardiac hypertrophy [7] . Filamin A (FLNA), the most widely expressed and abundant member of the filamin family of F-actin cross-linking proteins, is a critical mechanosensing element [8] , [9] that is essential for mechanoprotection, stretch-activated channel regulation, and the integration of distant parts of the cell to maintain the mechanical coherence of the cytoplasm [10] , [11] , [12] . FLNA is a homodimer of elongated subunits, each composed of an amino (N)-terminal actin-binding domain (ABD) followed by 24 Ig-like repeats segmented into two rod domains by ‘hinges’ ( Fig. 1a ) [13] , [14] . The second rod domain (repeats 16-23 or rod-2) contains the majority of binding sites for numerous and diverse cellular partners including signalling molecules and plasma membrane embedded proteins [13] , [15] . Structural studies of rod-2 have revealed that its partner-binding sites on repeats 19 and 21 are hidden by a β sheet designated strand A of repeats 18 and 20, respectively. In contrast to rod-1, the rod-2 Ig repeats overlap to form a more compact structure [16] , [17] , [18] , [19] , [20] . This architecture provides a basis for physiologically relevant forces to induce a conformational change in FLNA rod-2 that can expose these cryptic binding sites, particularly the integrin binding site on repeat 21 (refs 8 , 9 , 15 , 21 ). In vitro studies have experimentally documented such changes [8] , [21] . 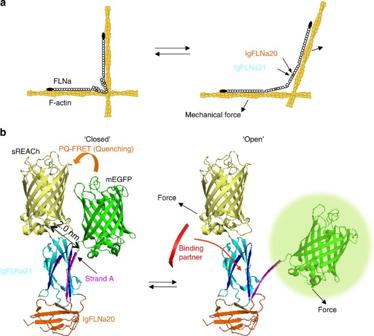Figure 1: The FLNA repeat 21-conformation sensor. (a) Model of FLNA crosslinking F-actin showing how its molecular conformation is altered by mechanical forces. FLNA interacts with F-actin through its N-terminal ABD and repeat 10 of rod-1 segment. This posits the rod-2 domain and the self-association site at the vertex of the crosslink where actin filament displacement can linearize the rod-2 domain. (b) Structure of FLNA repeats 20-21 (Protein Data Bank 2J3S) showing how strand A of repeat 20 auto-inhibits the partner-binding site on repeat 21 and how mechanical force displaces repeat 20 strand A to expose the 21 partner-binding site. The hypothetical location of mEGFP (donor) and sREACh (quencher) on the open and closed conformation of repeats 20-21 is shown. In the non-stressed state (left), the two fluorophores are in close proximity and the fluorescence of mEGFP is quenched by sREACh (or lifetime of mEGFP is shortened). When force opens the cryptic binding site (right), the probes move apart (PQ-FRET efficiency decreases and the fluorescence intensity of mEGFP increases or its lifetime becomes longer). Figure 1: The FLNA repeat 21-conformation sensor. ( a ) Model of FLNA crosslinking F-actin showing how its molecular conformation is altered by mechanical forces. FLNA interacts with F-actin through its N-terminal ABD and repeat 10 of rod-1 segment. This posits the rod-2 domain and the self-association site at the vertex of the crosslink where actin filament displacement can linearize the rod-2 domain. ( b ) Structure of FLNA repeats 20-21 (Protein Data Bank 2J3S) showing how strand A of repeat 20 auto-inhibits the partner-binding site on repeat 21 and how mechanical force displaces repeat 20 strand A to expose the 21 partner-binding site. The hypothetical location of mEGFP (donor) and sREACh (quencher) on the open and closed conformation of repeats 20-21 is shown. In the non-stressed state (left), the two fluorophores are in close proximity and the fluorescence of mEGFP is quenched by sREACh (or lifetime of mEGFP is shortened). When force opens the cryptic binding site (right), the probes move apart (PQ-FRET efficiency decreases and the fluorescence intensity of mEGFP increases or its lifetime becomes longer). Full size image Here we engineered a novel photoquenching fluorescence resonance energy transfer (PQ-FRET)-based FLNA sensor cassette that reports on this conformational change in cells ( Fig. 1b ). We demonstrate that full-length FLNA containing the FRET pair cassette is responsive to contractile force exerted by myosin embedded in actin networks in vitro . In living cells, time-lapse ratio imaging reveals that the FLNA sensor reports both spatial and temporal changes in FLNA conformation. Moreover, we show that ligands for FLNA repeat 21 induce molecular unfolding of that domain both in vitro and in vivo . These data confirm that FLNA-mediated mechanotransduction occurs in motile cells. Construction and characterization of FLNA PQ-FRET probes To detect the conformation changes of FLNA in cells, we constructed and inserted into the rod-2 segment of FLNA a genetically encoded PQ-FRET-based sensor. This sensor was composed of monomeric enhanced GFP (mEGFP) and a FRET fluorescence quencher, sREACh ( Fig. 1 ) that were separated by FLNA Ig repeats 20 and 21. We reasoned that ‘opening’ or dissociation of strand A of Ig-repeat 20 from its binding position on Ig-repeat 21 would increase the fluorescence emission of the sensor by moving sREACh away from mEGFP ( Fig. 1b ). sREACh is a nonfluorescent yellow fluorescent protein mutant with high absorbance that well overlaps with the emitted fluorescence of mEGFP, making sREACh an efficient quencher ( Supplementary Figs 1 and 2 ) [22] , [23] . To test this idea, we expressed, purified and assessed PQ- FRET pair constructs mEGFP and sREACH separated by various FLNA Ig repeats. Attachment of sREACh to the C terminus of mEGFP diminishes the fluorescence emission of mEGFP by 73±3% ( Fig. 2d ) whereas the insertion of one or more linear FLNA repeats between this FRET pair prevented quenching ( Fig. 2b ). Critically, an insertion of FLNA repeats 20-21 between the sensor pair reconstituted quenching: mEGFP fluorescence intensity was diminished by 44±5%, indicating that the 20-21 repeats position their ends and hence, the probes near one another ( Figs 1 and 2d ). We next added a TEV protease site after mEGFP to test if cleavage could relieve quenching ( Fig. 2 and Supplementary Fig. 1 ). Insertion of the cleavage site after mEGFP in the PQ-FRET probes slightly diminished the ability of the sREACh to quench, presumably by increasing the gap between them. However, mEGFP fluorescence further increased after cleavage of this linker sequence ( Supplementary Fig. 1 ). These data demonstrate that the PQ-FRET cassette linked with repeats 20-21 can detect conformational changes, whereas those linked with repeats 1-2, or lacking a linker, can serve as control standards that emit minimum or maximum mEGFP fluorescence, respectively. These sensor cassettes were Ca 2+ insensitive and responded proportionally to pH, validating them as intracellular sensors for different ionic environments ( Supplementary Fig. 3 ). Control probes with repeats 1-2, or without a linker, when they are embedded into full-length FLNA molecule, showed no change in FRET in vitro and in cells as described below. 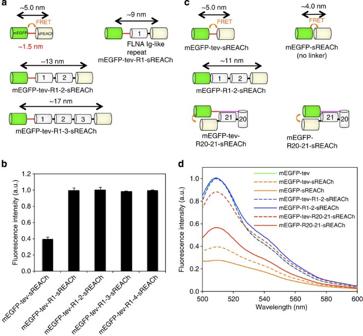Figure 2: Effect of insertions between mEGFP and sREACh on their FRET. (a,c) Schematic representation of fluorescence protein probes tested in this experiment. TEV protease recognition sequence (ENLYFQ) is indicated in red line. The strand A of repeat 20 is indicated in magenta. (b) Addition of a single FLNA Ig repeat between mEGFP and sREACh is sufficient to obliterate their FRET. Excitation was set at 458 nm and the emissions of mEGFP were measured at 511 nm. Error bars represent s.d. (n=3). (d) Removal of TEV protease recognition site (tev) increases FRET efficiency of mEGFP-tev-sREACh and EGFP-tev-R20-21-sREACh, but not that of mEGFP-tev-R1-2-sREACh. The emission spectrum is shown for excitation at 458 nm. Fluorescence intensities inbanddwere normalized to protein concentration and are given in arbitrary units (a.u.). Figure 2: Effect of insertions between mEGFP and sREACh on their FRET. ( a , c ) Schematic representation of fluorescence protein probes tested in this experiment. TEV protease recognition sequence (ENLYFQ) is indicated in red line. The strand A of repeat 20 is indicated in magenta. ( b ) Addition of a single FLNA Ig repeat between mEGFP and sREACh is sufficient to obliterate their FRET. Excitation was set at 458 nm and the emissions of mEGFP were measured at 511 nm. Error bars represent s.d. ( n =3). ( d ) Removal of TEV protease recognition site (tev) increases FRET efficiency of mEGFP-tev-sREACh and EGFP-tev-R20-21-sREACh, but not that of mEGFP-tev-R1-2-sREACh. The emission spectrum is shown for excitation at 458 nm. Fluorescence intensities in b and d were normalized to protein concentration and are given in arbitrary units (a.u.). Full size image FLNA binds F-actin through a high-affinity actin-binding domain and a low-affinity rod-1 segment (repeats 1-15) allowing force imposed on F-actin networks to concentrate at the rod-2 segment ( Fig. 1 ) [15] , [16] . Guided by this model, we inserted the sensor cassettes at two different locations of full-length FLNA molecules in the hope that force would efficiently transmit to the sensor while preserving the integrity and functionality of native FLNA molecules ( Supplementary Fig. 4 ). For example, the 20-21 sensor cassette was linked between repeat 17 and 22 of FLNA (repeats 18-21 were replaced with mEGFP-20-21-sREACh) because the: (1) probe contains four domains each of which has the similar size to each Ig repeat (two fluorophores and two Ig repeats, Supplementary Fig. 4b ) and; (2) N-terminal of repeat 19 is close to carboxy (C)-terminal of repeat 20 ( Supplementary Fig. 4c ) and this configuration is similar to the probe ( Supplementary Fig. 4b ). Since this probe responded best to mechanical strain in cells, all sensor cassettes were inserted at this position unless otherwise stated. The FLNA conformation sensor having repeats 20-21 inserted between the FRET pair was designated as FLNA-CS(20-21). FRET-FLIM imaging of FLNA conformation sensor in living cells Since FRET shortens the mEGFP donor lifetime in concentration-independent manner [24] , we anticipated that fluorescence lifetime imaging microscopy (FLIM)-FRET would be useful to visualize conformational changes of the FLNA probe in living cells. The probes were successfully expressed in COS-7 cells and the lifetime of mEGFP changed as expected ( Fig. 3 ). The wider distribution of lifetime between minimum and mean lifetime with FLNA-CS(20-21) suggests that there is more alterations in the lifetime of the donor in the confirmation sensitive probe compared with the lifetime of the donor itself and those of the control probes in living cells. However, the long acquisition times (2–3 min) required in FLIM measurements, limit its utility for monitoring dynamic events during cell protrusion and migration. 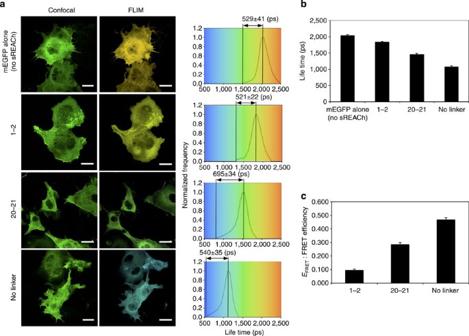Figure 3: FLIM-FRET study of FLNA-CS expressed in live COS-7 cells. (a) COS-7 cells were transfected with pFLAG-FLNA-CS with (repeats 1-2 or 20-21) or without linker between mEGFP and sREACh (Supplementary Fig. 4, without mCherry), or without sREACh and were used to acquire mEGFP intensity (confocal) and lifetime (FLIM) images. Bar, 20 μm. The lifetime distributions are shown for representative cells expressing FLNA-CS. The results of the fluorescence lifetime analysis are summarized inbandc. Error bars represent s.d. (n=3). FRET efficiency (EFRET) was calculated from EFRET=1−τDA/τDwhereτDAis the lifetime of the donor (mEGFP) in the presence of quencher (sREACh) andτDis the average lifetime of the donor in the absence of quencher. Figure 3: FLIM-FRET study of FLNA-CS expressed in live COS-7 cells. ( a ) COS-7 cells were transfected with pFLAG-FLNA-CS with (repeats 1-2 or 20-21) or without linker between mEGFP and sREACh ( Supplementary Fig. 4 , without mCherry), or without sREACh and were used to acquire mEGFP intensity (confocal) and lifetime (FLIM) images. Bar, 20 μm. The lifetime distributions are shown for representative cells expressing FLNA-CS. The results of the fluorescence lifetime analysis are summarized in b and c . Error bars represent s.d. ( n =3). FRET efficiency (E FRET ) was calculated from E FRET =1− τ DA / τ D where τ DA is the lifetime of the donor (mEGFP) in the presence of quencher (sREACh) and τ D is the average lifetime of the donor in the absence of quencher. Full size image Construction of an intensity-based FLNA PQ-FRET sensor To capture the rapid dynamics of the biosensor activities in high resolution, we used intensity-based ratiometric FRET [25] , [26] . The signal from the PQ-FRET probe depends on not only conformational changes of the probe but also its local concentration. Therefore, we attached mCherry to the N- or C-terminal end of FLNA ( Supplementary Fig. 4 ) as an internal control to normalize localized probe concentration because of its excellent stability and ease of quantified detection without interfering with mEGFP in our microscopic system ( Supplementary Fig. 2 ). The ratio of the two fluorophores (mEGFP/mCherry) thus reflects the liberation of the quenching group or conformational changes of the sensor. These probes retained F-actin gelation activity, the intrinsic fluorescence characteristics of native FLNA ( Supplementary Fig. 5 ), and distributed with endogenous FLNA in cytosol without altering cell morphology ( Supplementary Figs 6 and 7 ). In addition, negligible cross talk (bleed through) occurred between the mEGFP and mCherry signals, and the fluorescence of sREACh is low ( Supplementary Figs 2 and 6 ), simplifying image analysis ( Supplementary Table 1 ). Unfolding of purified FLNA-CS(20-21) by myosin in vitro We reconstituted homogeneous actomyosin networks crosslinked by recombinant FLNA-CSs in sealed chambers constructed from a gelsolin-coated coverslip and glass slide ( Fig. 4a ) [27] . We measured fluorescent intensities of mEGFP and mCherry using spinning-disk microscopy and plotted their ratio ( Fig. 4d,e ). The donor fluorescence intensity of FLNA-CS(20-21), embedded in F-actin networks, increased when myosin was added. This result indicates a lowering of donor energy transfer as the FRET pairs move further apart due to increasing myosin-based contractility, whereas control protein constructs were insensitive ( Fig. 4e ). To inhibit myosin contraction, we used a non-hydrolyzable ATP analogue ATP-γS, because more specific myosin inhibitors interfere with our FRET measurements [28] , [29] . Replacement of ATP with its non-hydrolyzable analogue reduced donor fluorescent intensity of FLNA-CS(20-21) ( Fig. 4e ), indicating that the FRET change is not simply due to myosin-mediated actin crosslinking. These results validate the probe as a mechanosensor. 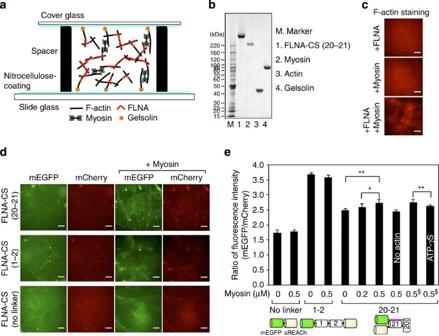Figure 4: Myosin-dependent conformational changes of purified FLNA-CS in actin networks. (a) Actin networks crosslinked with FLNA-CS are internally stressed by myosin motors. Actin filaments are anchored to glass surface through gelsolin coated on the surface. (b) Coomassie blue stain of SDS–PAGE gel of purified proteins used in this study. (c) 10 μM F-actin, crosslinked with 0.1 μM FLNA or not, was internally stressed by 0.5 μM myosin. F-actin is stained with Alexa Fluor 568 phalloidin. (d) Fluorescence images of mCherry-FLNA-CS (0.1 μM) embedded in actin filaments (10 μM) in the presence or absence of myosin (0.5 μM). Ratio of fluorescence intensities of mCherry and mEGFP was calculated and plotted ine. Scale bar, 10 μm. (e) Error bars represent s.d.,n≥4 independent experiments. §These two experiments were independently performed and compared. Statistical significance was determined by a two-tailedt-test (*P<0.05, **P<0.005). Figure 4: Myosin-dependent conformational changes of purified FLNA-CS in actin networks. ( a ) Actin networks crosslinked with FLNA-CS are internally stressed by myosin motors. Actin filaments are anchored to glass surface through gelsolin coated on the surface. ( b ) Coomassie blue stain of SDS–PAGE gel of purified proteins used in this study. ( c ) 10 μM F-actin, crosslinked with 0.1 μM FLNA or not, was internally stressed by 0.5 μM myosin. F-actin is stained with Alexa Fluor 568 phalloidin. ( d ) Fluorescence images of mCherry-FLNA-CS (0.1 μM) embedded in actin filaments (10 μM) in the presence or absence of myosin (0.5 μM). Ratio of fluorescence intensities of mCherry and mEGFP was calculated and plotted in e . Scale bar, 10 μm. ( e ) Error bars represent s.d., n ≥4 independent experiments. §These two experiments were independently performed and compared. Statistical significance was determined by a two-tailed t -test (* P <0.05, ** P <0.005). Full size image Conformational changes of FLNA-CS by a high-affinity ligand A high-affinity FLNA peptide ligand derived from the GPIbα cytoplasmic tail of the von-Willebrand Factor receptor has been reported to bind repeat 21 of FLNA in the absence of force [19] , [21] , [30] , [31] . We therefore determined if this peptide could induce the conformational change in the PQ-FRET sensor in FLNA-CS in vitro and in vivo . As expected, the GPIbα peptide markedly increased the fluorescent intensity of mEGFP linked to sREACh within the repeat 20-21 construct in a dose-dependent manner, whereas a β-integrin peptide emitted a much weaker signal ( Supplementary Table 2 and Supplementary Fig. 8 ). Time-lapse ratio images (mEGFP/mCherry) using FLNA-CS expressed in COS-7 and HEK-293 cells demonstrated that a cell-permeable GPIbα peptide (TAT-GPIbα) increased the relative fluorescent intensity of mEGFP when FLNA repeats 20-21 were inserted between the quenching pair. In contrast, FLNA-CS linked with repeats 1-2 or lacking a linker were insensitive to TAT-GPIbα peptide, and therefore, used as a standard for maximum and minimum ratio values in the scale, respectively ( Fig. 5 and Supplementary Fig. 9a and Supplementary Movies 1 and 2 ). As a control, we tested a GPIbα peptide mutated at critical amino acid residues for FLNA-binding ( Supplementary Table 2 ). This peptide did not unfold the auto-inhibition site on repeat 21 in vitro or in vivo ( Fig. 5 ). 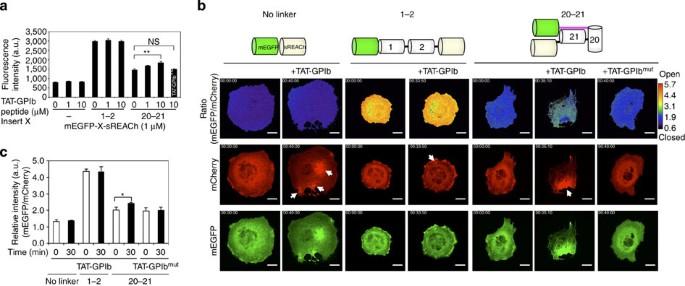Figure 5: A cell-permeable high-affinity ligand (TAT-GPIbα) for repeat 21 of FLNA induces conformational changes in the FLNA PQ-FRET probe (FLNA-CS) expressed in COS-7 cells. (a) Effect of increasing amounts of TAT-GPIbα peptide (0–10 μM) or TAT-GPIbα mutant peptide (10 μM) on the fluorescence intensity of purified mEGFP-sREACh constructs containing no linker, linked together with FLNA repeats 1-2, or linked together with repeats 20-21 (1.0 μM each). Fluorescence was measured in a microplate reader with excitation/emission wavelengths of 458/511 nm (mEGFP). (b) Fluorescence images of mCherry and mEGFP of FLNA-CS expressed in COS-7 cells before and after treatment with TAT-peptides. Ratio images and ratio colour scale (mEGFP/mCherry) were generated using Ratio Plus plugin (ImageJ). The cells were treated with 100-μM cell-permeable TAT-GPIbα peptide or TAT-GPIbα mutant peptide. Arrows highlight foci induced by the cell-permeable TAT-GPIbα peptide. Note that the ratio values at the foci are not quantitative because the fluorescence intensity was saturated. Scale bar, 20 μm. The corresponding movies are shown inSupplementary Movie 1. (c) The ratio of fluorescence intensities of mEGFP versus mCherry are plotted before and after treatment with the cell-permeable peptides. Error bars represent s.d. (n=3). *P<0.05, **P<0.005; NS, not significant by a two-tailedt-test. Figure 5: A cell-permeable high-affinity ligand (TAT-GPIbα) for repeat 21 of FLNA induces conformational changes in the FLNA PQ-FRET probe (FLNA-CS) expressed in COS-7 cells. ( a ) Effect of increasing amounts of TAT-GPIbα peptide (0–10 μM) or TAT-GPIbα mutant peptide (10 μM) on the fluorescence intensity of purified mEGFP-sREACh constructs containing no linker, linked together with FLNA repeats 1-2, or linked together with repeats 20-21 (1.0 μM each). Fluorescence was measured in a microplate reader with excitation/emission wavelengths of 458/511 nm (mEGFP). ( b ) Fluorescence images of mCherry and mEGFP of FLNA-CS expressed in COS-7 cells before and after treatment with TAT-peptides. Ratio images and ratio colour scale (mEGFP/mCherry) were generated using Ratio Plus plugin (ImageJ). The cells were treated with 100-μM cell-permeable TAT-GPIbα peptide or TAT-GPIbα mutant peptide. Arrows highlight foci induced by the cell-permeable TAT-GPIbα peptide. Note that the ratio values at the foci are not quantitative because the fluorescence intensity was saturated. Scale bar, 20 μm. The corresponding movies are shown in Supplementary Movie 1 . ( c ) The ratio of fluorescence intensities of mEGFP versus mCherry are plotted before and after treatment with the cell-permeable peptides. Error bars represent s.d. ( n =3). * P <0.05, ** P <0.005; NS, not significant by a two-tailed t -test. Full size image Spatio–temporal regulation of FLNA-CS unfolding in cells We reacted COS-7 and HEK-293 cells transfected with the three FLNA-CS probes with phorbol 12-myristate 13-acetate (PMA) to induce cell spreading and migration [32] , [33] . These cell lines were chosen because of their ease of transfection. The large size of COS-7 cells facilitates visualizing the molecular dynamics of a given protein in the cytosol. Since fluorescence intensity decreases when a lower-power objective lens is used, and different lenses may impact on mEGFP/mCherry ratios, we used the same high-power (× 60) objective lens throughout our experiments. To monitor multiple cells, we used HEK-293 cells, which are relatively small. We found that the rod-2 domain of FLNA opens in specific cellular locations following cell stimulation with PMA ( Fig. 6 and Supplementary Movies 3–5 ). Quantified measurements of relative intensities in different regions of cells as a function of time revealed that maximal opening of repeat 21 occurs 5–10 min after the addition of PMA and that unfolding occurs predominantly at the cell edge; the relative intensity of the FLNA-CS (20-21) probe increased by 11% at the cell edge (2.40±0.03 to 2.64±0.08, mean±s.d. (circled regions 7 and 8 in Fig. 6b,c ). No ratio change was observed in cells transfected with constructs containing no linker or repeats 1-2 between the FRET pair ( Fig. 6 and Supplementary Fig. 9 and Supplementary Movies 3 and 4 ), endorsing the methodology. 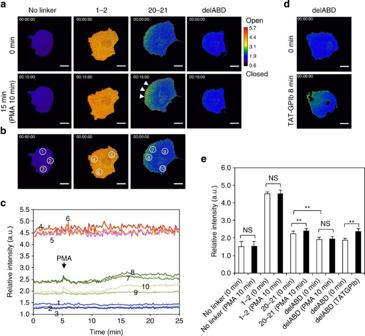Figure 6: Conformational changes in the FLNA-CS(20-21) probe expressed in COS-7 cells require binding to the actin cytoskeleton. (a) Spatial conformational changes in FLNA-CSs expressed in COS-7 cells following PMA treatment. Scale bar, 20 μm. The corresponding movies are shown inSupplementary Movie 3. (b–e) Quantification of spatial conformational changes in the FLNA-CSs probe expressed in COS-7 cells. Intensities of different regions (circled inb) of the ratio images were quantified and plotted as a function of time (c). COS-7 cells expressing FLNA-CS(20-21) lacking its ABD before and after treatment with cell-permeable TAT-GPIbα peptide (d). The corresponding movies are shown inSupplementary Movie 6. Average intensities of three independent ratio images (whole cells) before and after PMA stimulation were quantified and plotted (e). Error bars represent s.d. (n=3). **P<0.005; NS, not significant by a two-tailedt-test. Figure 6: Conformational changes in the FLNA-CS(20-21) probe expressed in COS-7 cells require binding to the actin cytoskeleton. ( a ) Spatial conformational changes in FLNA-CSs expressed in COS-7 cells following PMA treatment. Scale bar, 20 μm. The corresponding movies are shown in Supplementary Movie 3 . ( b – e ) Quantification of spatial conformational changes in the FLNA-CSs probe expressed in COS-7 cells. Intensities of different regions (circled in b ) of the ratio images were quantified and plotted as a function of time ( c ). COS-7 cells expressing FLNA-CS(20-21) lacking its ABD before and after treatment with cell-permeable TAT-GPIbα peptide ( d ). The corresponding movies are shown in Supplementary Movie 6 . Average intensities of three independent ratio images (whole cells) before and after PMA stimulation were quantified and plotted ( e ). Error bars represent s.d. ( n =3). ** P <0.005; NS, not significant by a two-tailed t -test. Full size image FLNA-CS(20-21) lacking the ABD, which retains sensitivity to TAT-GPIbα-binding, diffusely localizes in the cytoplasm, and the intensity of its ratio image was lower than that of full-length FLNA-CS(20-21) and was not changed by PMA stimulation ( Fig. 6 ). In elongated cells, unfolded FLNA-CS(20-21) localizes mainly at the cell ends ( Supplementary Fig. 10 and Supplementary Movie 7 ). Depolymerization of actin filaments with latrunculin A closed the mechanosensing site of FLNA localized at these regions ( Supplementary Fig. 10 and Supplementary Movie 7 ). We transfected our probes into mouse embryonic fibroblast (MEF) cells and stimulated them with lysophosphatidic acid (LPA) to activate the well-established signalling pathway to myosin contraction downstream involving Rho/Rho-kinase [34] . To optimize transfection efficiency, the plasmid vector was switched, and a different transfection reagent used (see Methods). Consistent with the above results, no ratio change was observed in MEF cells transfected with constructs containing no linker or repeats 1-2 between the FRET pair ( Fig. 7 and Supplementary Movie 7 ). Upon LPA stimulation, MEF cells transfected with the FLNA-CS(20-21) probe contracted, and the FRET ratio (mEGFP/mCherry) increased. Relative changes of ratio in different regions of cells as a function of time showed that maximal FLNA probe opening of repeat 21 occurred ~10 min after the addition of LPA and that unfolding was restricted to protruding regions where the relative intensity of the FLNA-CS (20-21) probe increased by 6–10% ( Fig. 7 and Supplementary Movie 7 ). We used the Rho-kinase inhibitor, Y27632, to suppress myosin contraction [35] . Pretreatment of MEF cells with Y27632 inhibited LPA-induced opening of FLNA-CS(20-21) ( Supplementary Fig. 11 and Supplementary Movie 9 ). 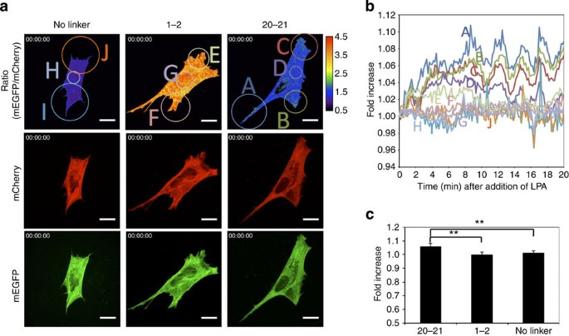Figure 7: LPA-induced myosin contraction increases conformational changes in the FLNA-CS(20-21) probe expressed in MEF cells. (a) Spatial conformational changes in FLNA-CSs expressed in MEF cells following LPA (1 μM) treatment. Scale bar, 20 μm. The corresponding movies are shown inSupplementary Movie 8. (b,c) Quantification of spatial conformational changes in the FLNA-CSs probe expressed in MEF cells stimulated with LPA. Intensities of different regions (circled ina) of the ratio images were quantified, normalized (relative to before stimulation) and plotted as a function of time (b). Changes of average intensities of 10 independent ratio images before and after (15 min) LPA stimulations were quantified and plotted (c). Error bars represent s.d. (n=10). **P<0.005 by a two-tailedt-test. Figure 7: LPA-induced myosin contraction increases conformational changes in the FLNA-CS(20-21) probe expressed in MEF cells. ( a ) Spatial conformational changes in FLNA-CSs expressed in MEF cells following LPA (1 μM) treatment. Scale bar, 20 μm. The corresponding movies are shown in Supplementary Movie 8 . ( b , c ) Quantification of spatial conformational changes in the FLNA-CSs probe expressed in MEF cells stimulated with LPA. Intensities of different regions (circled in a ) of the ratio images were quantified, normalized (relative to before stimulation) and plotted as a function of time ( b ). Changes of average intensities of 10 independent ratio images before and after (15 min) LPA stimulations were quantified and plotted ( c ). Error bars represent s.d. ( n =10). ** P <0.005 by a two-tailed t -test. Full size image Finally, we investigated spatio–temporal changes of FLNA-CS(20-21) in MEF cells undergoing shape change and migration after starvation and stimulation with serum ( Supplementary Movie 10 ). Opening of FLNA-CS(20-21) was observed in the protruding regions of these cells, and opening of FLNA reversed as protrusive activity ceased. Although filamin is bound in stress fibres and mature adhesion sites, molecular opening was not observed in these areas. Maximum probe closing was observed when cells rounded due to the loss of adhesion or intracellular contraction (left upper panel in Supplementary Movie 10 ). Although open FLNA has a higher affinity for β-integrin tail than closed molecules [8] , [21] , we did not observe FLNA accumulation at focal adhesion sites or stress fibres and instead, found a broad distribution of the open probe in actively protruding cytoplasm. Mechanosensing molecules function to transmit and transduce force to regulate key biological processes such as focal adhesion formation, differentiation, growth and mechanosensing abnormalities and loss of mechanoprotection are implicated in disease processes [36] , [37] , [38] , [39] . Since mechanotransduction is mediated by changes in the structure of specific molecules in cells, spatio–temporal information on such conformational changes in cells and tissue is crucial. However, only limited methodology is available to monitor mechanotransduction events in general and the only currently available techniques to accomplish this task in vivo is FRET [40] . Furthermore, insufficient structural information concerning the limited number of molecules identified as mechanosensor elements limits construction of useful FRET probes [6] , [8] , [41] , [42] , [43] . In contrast, much information predicts that mechanotransduction in FLNA is triggered by conformational changes that expose the cryptic binding site of repeat 21. Hence, our FRET pair was designed to unquench as the conformation of FLNA opens and reports positive fluorescence as opposed to conventional FRET where fluorescence would decrease. Therefore, when most of the FLNA molecules are dormant (closed), the signal from the probe is low, alleviating signal-to-noise complications in detection within a high background. Because of this low background, we were able to detect an ~11% increase of relative intensity of mEGFP in cells expressing FLNA-CS(20-21) after PMA stimulation. Although an FLNA-based probe has been previously used to reveal mechanotransduction, it has not been applied to cell dynamics and movement [44] , [45] . This probe contains a conventional FRET pair (Cerulean/Venus) inserted at position 1,000 in the FLNA molecule. This positions it within repeat 8 and between two F-actin-binding sites (N-terminal ABD and repeat 10 (refs 16 , 46 ). For this probe to report, repeat 8 must be unfolded. Unfolding of an Ig repeat requires higher forces (>30 pN) than those which open the repeat domain pairing between repeat 20 and 21 (2–5 pN) [21] , [47] , [48] . It is not clear if such repeat unfolding occurs in living cells. In addition, the biological meaning of unfolding repeat 8, if any, has not been documented. The atomic structures of repeats 20-21 of FLNA are well defined, and force-induced ligand binding to repeat 21 has been demonstrated [8] , [17] , [21] . In this study, using our mechanosensor probe, we documented temporal and spatial conformational changes in this domain in living cells. Myosin-dependent opening of FLNA-CS(20-21) was observed only in protruding regions of cells, and not in stress fibres or focal adhesions. Opening in focal adhesions was predicted, because the open form of FLNA has a higher affinity for the β-integrin tail [8] , [21] . Since previous studies showed that FLNA competes with talin and is a negative regulator of integrin activation [49] , [50] , our findings suggest that open FLNA does not translocate to focal adhesion, but rather binds to integrins in protruding cell regions, which are subsequently delivered to talins at focal adhesion. In addition to β-integrins, FLNA repeat 21 also interacts with migfilin and a large number of possible partners (SEK1, JNK1 and so on) whose interactions have been delimited to larger regions of the FLNA molecule that include repeat 21 (refs 15 , 49 , 51 , 52 ). Since the affinity of β-integrin tail for the CD pocket in repeat 21, when covered with strand A of repeat 20 in an unstressed state, is insufficient to dissociate strand A, force can regulate this interaction. High-affinity ligands, such as the GPIbα tail can also bind FLNA’s repeat 21 in the absence of force, and induce a conformational change detected by FLNA-CS(20-21) [19] , [21] , [31] . Hence, PMA-stimulated unfolding of the sensor could be induced by ligand binding or by force. However, expression of FLNA-CS(20-21) without its N-terminal ABD significantly reduced the basal level of fluorescent signal in cells and made the sensor unresponsive to PMA stimulation. In addition, the conversion of FLNA-CS(20-21) to the open form in MEF cells is LPA-dependent and suppressed with a Rho-kinase inhibitor. These data indicate that ligand binding to repeat 21 requires myosin-mediated contractile force transmitted through the actin cytoskeleton. The loss of signal from labelled FLNA lacking its actin-binding domain further implies that FLNA linked to actin filaments is prestressed, although, as suggested previously, its repeat 21 is not fully unfolded [53] . Although stress fibres are force-generating and tension-bearing structures [54] , FLNA-CS(20-21) was not converted to its open conformation in stress fibres, suggesting that three-dimensional orthogonal structure of FLNA/F-actin networks optimizes this conformational change in FLNA. Although FLNA molecules reside throughout the cytoplasm, in particular in F-actin-rich regions, the open FLNA configuration recognized by our probe localized strikingly at the dynamic protruding leading edges of activated cells. This finding is consistent with much known information about the structure of FLNA-F-actin complexes in different circumstances [16] , [55] . FLNA molecules in complexes composed of low FLNA-actin ratios in vitro (such as those we used to validate activation of the probe under myosin-induced contractile tension) and characteristic of the leading edge of motile cells reside at the vertices of orthogonal crosslinked actin networks (as depicted in Fig. 4 ). Exposed to force induced by myosin-based F-actin contraction or conceivably hydrostatic pressure [56] , such networks would be expected to deform in a manner that would open the C-terminal domains of FLNA. The resulting accessibility of those domains to many binding partners of FLNA relevant to cell signalling is consistent with the leading cell edge being a region where many if not most intracellular signalling reactions occur. In contrast, at high FLNA-actin ratios in vitro or when the FLNA is bound to F-actin in stress fibre bundles, at the contracted back ends of polarized cells or in dense complexes of cell adhesion structures, FLNA molecules would predictably be compressed, and their C-terminal partner-binding domains closed. PQ-FRET should be applicable to study any biomaterial capable of signal emission in response to inter- or intramolecular dissociation [57] . It may be useful for high-throughput screening for molecules or drugs that regulate mechanotransduction and protein conformational changes as demonstrated here with the synthetic peptide derived from the GPIbα tail. In conclusion, using a novel and defined FLNA-based mechanosensing probe, we found that opening of the integrin binding site of FLNA occurs at actively protruding regions of moving cells but not at retracting regions, focal adhesions or stress fibres. These results indicate that mechanical forces exerted in cortical orthogonal actin networks to FLNA recruits signalling molecules to protruding regions. Synthetic peptides and chemicals Synthetic peptides ( Supplementary Table 2 ) were purchased from Peptide 2.0 (>95% purity) and dialyzed against phosphate-buffered saline (PBS) using Micro Float-A-Lyzer (Spectrumlabs). Other chemicals were purchased from Sigma unless otherwise specified. Plasmid construction pFASTBAC-HTb (Invitrogen, San Diego, CA, USA) vector for protein expression in insect cells was modified by the insertion of cDNA encoding EGFP, sREACh and FLNA domains using conventional molecular biology techniques. To engineer pFASTBAC-HTb-mEGFP-tev and pFASTBAC-HTb-mEGFP, cDNA encoding mEGFP was amplified by PCR using pEGFP-C1 (Clontech) mutated at A206K as the template, the forward primer, 5′- CATG CCATGG TGAGCAAGGGCGAG -3′, containing a NcoI site, and the reverse primers, 5′- CG GGATCC CTGAAAATACAGGTTTTCGATCCCGGCGGCGG -3′, containing a BamHI site and encoding TEV cleavage site (ENLYFQ/G) or 5′- CG GGATCC GATCCCGGCGGCGGTC -3′, containing a BamHI site without encoding TEV cleavage site. The amplified fragment was purified, NcoI / BamHI -digested and ligated into NcoI / BamHI sites in the pFASTBAC-HTb vector. To generate pFASTBAC-HTb-mEGFP-tev--sREACh and pFASTBAC-HTb-mEGFP--sREACh, cDNA encoding sREACh was amplified by PCR using pCAG-sREACh-Actin (Addgene [23] ) as the template, the forward primer, 5′- CGC GTCGAC AAGGGCGAGGAGCTGTTC -3′ containing a SalI site, and the reverse primer, 5′- GC TCTAGA TCAGATCCCGGCGGCGGTC -3′, containing a XbaI site. The amplified fragment was purified, SalI / XbaI -digested and ligated into SalI / XbaI sites in pFASTBAC-HTb-mEGFP-tev and pFASTBAC-HTb-mEGFP vectors. To engineer pFASTBAC-HTb-mEGFP-tev-sREACh and pFASTBAC-HTb-mEGFP-sREACh, cDNA encoding sREACh was amplified by PCR using pCAG-sREACh-Actin (Addgene) as the template, the forward primer, 5′- CG GGATCC GTGAGCAAGGGCGAGGAG -3′, containing BamHI site, and the reverse primer, 5′- GC TCTAGA TCAGATCCCGGCGGCGGTC -3′, containing XbaI site. To insert cDNA encoding FLNA Ig domains into pFASTBAC-HTb-mEGFP-tev and pFASTBAC-HTb-mEGFP vectors, FLNA Ig domains were amplified by PCR using primers containing BamHI site (forward primer) and SalI site (reverse primer) and the amplified fragments were ligated into BamHI/SalI sites in the vectors. pmCherry-FLNA was engineered using pmCherry-C1 (Clontech). Briefly, the N-terminal FLNA domain (1–154 aa) was subcloned into BglII/EcoRI sites of pmCherry-C1 by PCR using pEGFP-FLNA as the template, the forward primers 5′- CG GGATCC ATGAGTAGCTCCCACTCTC -3′, and the reverse primer 5′- G GAATTC AGGGCATGGAGATGGAG -3′. pmCherry-FLNA was generated by inserting a fragment of FLNA cDNA digestested out from pFASTBAC-FLNA vector with SalI and XbaI into pmCherry-FLNA(1–154). pFASTBAC-HTb-mCherry-FLNA was engineered from pFASTBAC-HTb. Briefly, cDNA encoding mCherry was amplified by PCR using pmCherry-C1 as the template, the forward primer, 5′- GA AGATCT ATGGTGAGCAAGGGCGAGG -3′, containing a BglII site, the reverse primer, 5′- CG GGATCC GAGTCCGGACTTGTACAGCTCGTCCA -3′, containing a BamHI site. The amplified fragments were purified, BglII / BamHI -digested and ligated into BamHI sites in the pFASTBAC-HTb vector to generate pFASTBAC-HTb-mCherry. The N-terminal FLNA domain (1–154 aa) was subcloned into BamHI/EcoRI sites of pFASTBAC-HTb-mCherry by PCR using pEGFP-FLNA as the template, the forward primers 5′- CG GGATCC ATGAGTAGCTCCCACTCTC -3′, and the reverse primer 5′- G GAATTC ACGTCACTTGGAAGGGGC -3′. pFASTBAC-HTb-mCherry-FLNA was generated by inserting a fragment of FLNA cDNA digested out from pFASTBAC-FLNA vector with SalI and XbaI into pFASTBAC-HTb-mCherry-FLNA(1–154). mCherry was also attached at the C-terminal of full-length FLNA as follows. First, cDNA encoding FLNA repeat 24 was amplified by PCR using pFASTBAC-FLNA as the template, the forward primer, 5′- CGGGATCCGCTGACGCCAGCAAGGTG -3′, the reverse primer, 5′- CTG GAGCTCTCTAGA GGC GCGGCCGC GGGGCACCACAACGCGG -3′, containing a SacI site (and NotI and XbaI sites). The amplified fragments were purified, EcoNI / SacI -digested and ligated into EcoNI/SacI sites in the pBluescript II (+)-FLNA( ClaI/XbaI ) vector that was generated by subcloning 3′ fragment of FLNA cDNA digested out from pFASTBAC-FLNA vector with ClaI and XbaI . cDNA encoding mCherry was amplified by PCR using pmCherry-C1 as the template, the forward primer, 5′- GAAT GCGGCCGC AATGGTGAGCAAGGGCGAGG -3′, containing a NotI site, the reverse primer, 5′- GC TCTAGA CTACTTGTACAGCTCGTCCATG -3′, containing XbaI site. The amplified fragments were purified, NotI / XbaI -digested and ligated into NotI / XbaI sites in the pBluescript II (+)-FLNA( ClaI/XbaI )-vector containing NotI and XbaI sites to generate pBluescript II (+)-FLNA( ClaI/XbaI )-mCherry vector. To engineer full-length FLNA constructs, FLNA repeats 18-21 were deleted and simultaneously SpeI and AflII sites were introduced between repeats 17 and 22, hinge-1 and repeat 16, or strand A of repeat 16 and repeat 23 using QuickChange Site-Directed Mutagenesis kit (Agilent Technologies, Santa Clara, CA, USA) in accordance with the manufacturer’s protocol. Briefly, the following primers were designed 5′- CACAGGTGACGAC ACTAGTCTTAAG GGCGACGCCCGCCG -3′ and 5′- CGGCGGGCGTCGCCCTTAAGACTAGTGTCGTCACCTGTG -3′, 5′- CCAGCAGACTTGG ACTAGTCTTAAG GCCCCGGAGAGGC -3′ and 5′- GCCTCTCCGGGGC CTTAAGACTAGT CCAAGTCTGCTGG -3′, or 5′- TGTCAATGGGCTGGAT ACTAGTCTTAAG GGGGACCCAGGCTT -3′ and 5′- AAGCCTGGGTCCCC CTTAAGACTAGT ATCCAGCCCATTGACA -3′. PCR was done on pBluescript II (+)-FLNA( ClaI/XbaI ). To introduce SpeI site at 5′ terminus of mEGFP of pFASTBAC-HTb-mEGFP, the forward primer, 5′- CATG CCATGG CAACTAGTATGGTGAGCAAGGGCG -3′, containing a NcoI site was used instead of 5′- CATG CCATGG TGAGCAAGGGCGAG -3′ described above. Likewise, AflII sites at 3′ terminus of sREACh of pFASTBAC-HTb-mEGFP-tev—sREACh was introduced using the reverse primer, 5′- GC TCTAGA CTTAAGCCCGGCGGCGGTCACTCT -3′, containing XbaI site instead of 5′- GC TCTAGA TCAGATCCCGGCGGCGGTC -3′ as described above. The cDNA encoding mEGFP-sREACh with or without FLNA Ig repeats were digested with SpeI and AflII and ligated into pBluescript II (+)-FLNA( ClaI/XbaI )-R17- SpeI/AflII -R22, pBluescript II (+)-FLNA( ClaI/XbaI )-H1- SpeI/AflII -R16, or pBluescript II (+)-FLNA( ClaI/XbaI )-R16stA- SpeI/AflII -R23. For some construct, mCherry was attached to the C-terminal of FLNA by inserting EcoNI / XbaI -digested fragment of pBluescript II (+)-FLNA( ClaI/XbaI )-mCherry into these constructs. The FLNA fragment containing the mEGFP-sREACh reporters were digested out with ClaI and XbaI and ligated into pFASTBAC-HTb-mCherry-FLNA, pmCherry-FLNA, and pFLAG-FLNA. Likewise, the mEGFP-sREACh reporters were inserted at position 1,000 as previously described [45] . To switch the CMV promoter of pFLAG-FLNA constructs to EF1α promoter, pBApo-EF1α Neo DNA (Takara) was digested with XbaI and calf intestinal alkaline phosphatase and ligated with fragments derived from the pFLAG-FLNA constructs digested with NheI and XbaI. pFASTBAC-HTb-Halo-mCherry was constructed by PCR. Briefly, cDNA encoding Halo-tag was amplified by PCR using pFN21A HaloTag CMV Flexi Vector (Promega) as the template, the forward primer, 5′- CATG CCATGG CAGAAATCGGTACTGG -3′, containing a NcoI site, and the reverse primer, 5′- GC GGATCC TCCACCGGAAATCTCCAGAGTAGACAGCCAGCGCGCGATC -3′, containing BamHI site. The amplified fragments were purified, NcoI / BamHI -digested and ligated into NcoI / BamHI sites in the pFASTBAC-HTb vector to generate pFASTBAC-HTb-Halo. Next, cDNA encoding mCherry was amplified by PCR using pmCherry-C1 as the template, the forward primer, 5′- GA AGATCT ATGGTGAGCAAGGGCGAGG -3′, containing a BglII site, and the reverse primer, 5′- CG GGATCC GAGTCCGGACTTGTACAGCTCGTCCA -3′, containing BamHI site. The amplified fragments were purified, BglII / BamHI -digested and ligated into BamHI sites in the pFASTBAC-HTb-Halo vector to generate pFASTBAC-HTb-Halo-mCherry. To generate pFASTBAC-HTb-Halo-mCherry-16-23-Avi, the cDNA fragment encoding IgFLNa16-23-Avi was digested out from pFASTBAC-HTb-16-23-Avi using BamHI and HindIII , and ligated into pFASTBAC-HTb-Halo-mCherry digested with BamHI and HindIII . The cDNA encoding the force sensor was inserted into pFASTBAC-HTb-Halo-mCherry-16-23-Avi using BspMI digestion of pBluescript II (+)-FLNA( ClaI/XbaI )-R17-EGFP-sREACh-R22. Expression and purification of recombinant protein Recombinant proteins were expressed using a Baculovirus Expression System (Invitrogen) in sf9 insect cells and purified [58] . A virus was generated with the BAC-TO-BAC system (Invitrogen). Sf9 cells were cultured in Sf-900 II SFM (Invitrogen) supplemented with 50 units ml −1 penicillin and 50 μg ml −1 streptomycin and used for virus amplification and protein expression. Forty-eight hours post infection, the cells were collected by centrifugation, washed with PBS and stored at −80 °C. The expressed proteins were purified by Ni-NTA affinity and gel filtration chromatography (Superose 12 and Superdex 200, GE Healthcare) [58] . In brief, the proteins were extracted from the Sf9 cells in lysis solution (20 mM sodium phosphate, pH 8.0, 100 mM NaCl, 20 mM imidazole,1 mM β-mercaptoethanol, 2 mM PMSF, 10 μg ml −1 aprotinin and 10 μg ml −1 leupeptin) at 4 °C. The extracts were centrifuged at 20,000 g for 30 min at 4 °C and loaded onto a Ni-NTA column (1 ml; QIAGEN). The column was washed with washing solution I (20 mM sodium phosphate, pH 8.0, 20 mM imidazole, 1 mM β-mercaptoethanol, 300 mM NaCl, 0.1% Triton X-100) followed by washing solution II (20 mM sodium phosphate, pH 8.0, 20 mM imidazole, 100 mM NaCl, 1 mM β-mercaptoethanol) and bound recombinant proteins were eluted with 20 mM sodium phosphate, pH 8.0, 200 mM imidazole, 1 mM β-mercaptoethanol. Purified proteins were concentrated using an Amicon Ultra-15 (Millipore) and gel-filtered on Superose 12 and Superdex 200 (10/300; GE Healthcare) columns pre-equilibrated with PBS. Full-length FLNA proteins containing the mEGFP-sREACh reporters were purified by ion-exchange and gel filtration chromatography [16] . In brief, protein extracts were prepared by suspending the Sf9 cells in a solution containing 10 mM Tris–HCl, pH 8.5, 100 mM NaCl, 1% Triton X-100, 10 mM EGTA, 1 mM EDTA, 5 mM 2-mercaptoethanol and a mixture of protease inhibitors (10 μg ml −1 each chymostatin, leupeptin and pepstatin and 1 mM phenylmethylsulfonyl fluoride). The cell lysates were centrifuged at 20,000 × g at 4 °C and the supernatant fluid was loaded onto a HiTrap Q column (5-ml column, GE Healthcare) pre-equilibrated with buffer solution QA8.5 (10 mM Tris–HCl, pH 8.5, 1 mM EDTA, 1 mM EGTA, 5 mM 2-mercaptoethanol, 0.02% Triton X-100). Proteins were eluted with a 100-ml linear gradient of 200–400 mM NaCl in the equilibrating buffer at a flow rate of 4 ml min −1 . Fractions containing recombinant FLNA-CS (eluting around 300 mM NaCl) were pooled and diluted 1:2 with QA8.5 solution containing the protease inhibitor mixture. Proteins in the pooled fractions were absorbed again onto a HiTrap Q column, and the column was washed with QA6.5 solution (10 mM PIPES-NaOH, pH 6.5, 1 mM EDTA, 1 mM EGTA, 5 mM 2-mercaptoethanol, 0.02% Triton X-100) containing 100 mM NaCl. Recombinant FLNA was eluted with a linear salt gradient (100 ml) from 100–400 mM NaCl in buffer QA6.5 at a flow rate of 4 ml min −1 . Fractions containing FLNA-CS (eluting around 200 mM NaCl) were pooled and concentrated using Ultrafree-15 (Biomax-50K, Millipore). FLNA-CS was further purified by Superose 6 (GE Healthcare) column chromatography with S6 solution (10 mM Tris–HCl, pH 7.4, 120 mM NaCl, 0.5 mM EGTA, 1 mM dithiothreitol). Isolated FLNA-CS was concentrated using Ultrafree-15, frozen in liquid nitrogen, and stored at −80 °C [16] , [58] . Protein concentration was measured by absorption at 280 nm using parameter calculated by ProtParam tool ( http://au.expasy.org/tools/protparam.html ) or 660-nm protein assay kit (Pierce). Recombinant protein was stored at −80 °C and thawed and clarified before use. F-actin gel point assay Gelation was determined using a miniature falling ball viscometer [59] . Actin polymerization was initiated by the addition of 24 μM unpolymerized actin in the presence or absence of different concentrations of FLNA-CS in buffer B (20 mM Tris–HCl, 100 mM KCl, 2 mM MgCl 2 , 0.5 mM EGTA, 0.5 mM ATP). The mixtures were immediately drawn into vertically positioned 100-μl capillary tubes (Fisher) and incubated at 25 °C for 60 min unless indicated otherwise. The time required for a 0.7-mm diameter stainless steel ball to fall 5 cm was measured [59] . Fluorometry Fluorescence intensities of purified proteins were measured by a fluorescence microplate reader (SpectraMax Gemini EM, Molecular Devices). Cell culture and expression of FLNA-CS in mammalian cells HEK-293 and COS-7 cells were trypsinized with 0.05% trypsin/EDTA for 5 min and centrifuged in PBS. The cells were resuspended in growth medium and placed on a Lab-Tek II chamber slide (Cat# 154534, Thermo Scientific: for scanning-disk microscopy) and Delta T culture dishes (Cat# 04200415C, Bioptechs, Butler, PA: for FLIM) coated with 0.1% (w/v) gelatin solution (G1393, Sigma-Aldrich) or 10 μg ml −1 fibronectin (F0895, Sigma-Aldrich) for overnight in a 5% CO 2 incubator at 37 °C. The cells were transfected with TransIT-LT1 (Mirus Bio) in accordance with manufacturers’ instructions 24 or 48 h before imaging. Three hours before imaging, growth medium were replaced with growth medium supplemented with 25 mM HEPES without phenol red. MEF cells were cultured on a Lab-Tek II chamber slide coated with 0.1% (w/v) gelatin. The growth medium was replaced with Opti-MEM (Life technologies) and the cells were transfected with TransIT-X2 (Mirus Bio). Twenty-hours post transfection, the medium was replaced with growth medium supplemented with 25 mM HEPES without serum and phenol red. In some experiments, transfected cells were treated with a pharmacological activator or inhibitor as indicated in the figure legends. Fluorescence lifetime microscopy FLIM was performed using a Becker & Hickl time correlated single photon counting (TCSPC) system with a Hamamatsu hybrid detector (model HPM-100-50; Hamamatsu Photonics) attached to the non-descanned detection light path on a Zeiss 710 laser-scanning confocal/multi-photon system with an upright Zeiss Examiner Z.1 stand. Two-photon excitation was achieved using a Chameleon Vision II laser (Coherent) to pump a mode-locked frequency-doubled Ti:Sapphire laser that provided 140-femtosecond pulses at a 80-Mhz repetition rate with an output power of 3 W at the peak of the tuning curve (800 nm). EGFP and sREACh fluorophores were used as a FRET pair for all of the FLIM-FRET measurements. The two-photon laser was set to 920 nm for excitation of the donor (EGFP). Fluorescence emission of EGFP fusion proteins was collected using a bandpass filter (500–550 nm) to limit detection to only the donor. Laser power was adjusted to 14% to give a mean photon count rate of the order 10 4 photons per second. For imaging live cells by FLIM, cells were plated in Delta T culture dish coated with 0.1% (w/v) gelatin solution. The dish and Zeiss W Plan-Apochromat 63x/1.0NA objective were heated using feedback control Bioptechs objective and stage heater. For fixed cells, transfected cells were cultured on a cover glass coated with 0.1% (w/v) gelation and fixed with 4% formaldehyde (EM grade, Electron Microscopy Sciences) in PBS for 20 min at 37 °C. The cells were rinsed with 20 mM Tris–HCl, pH 7.4, 150 mM NaCl and mounted in PermaFluor (Thermo Scientific). Fluorescence from fixed samples was collected with a Zeiss Plan-Apochromat 63x/1.40 NA Oil objective. Spinning-disk confocal microscopy and image acquisition Cells expressing PQ-FRET sensors were imaged using a spinning-disk confocal microscope: spinning-disk head (CSU-X1, Yokogawa), microscope stand (IX81, Olympus), 488 nm and 561 nm laser combiner (ALC, Andor Technology), EMCCD camera (iXon 897, Andor Technology), laser based focusing system (ZDC1, Olympus), objective (60 × /1.2 NA UPLSAPO 60XW water immersion lens, Olympus), image acquisition software (MetaMorph 7.7.7.0, Molecular Devices), stage top humidified chamber (INU-ZILCS-F1, Tokai Hit), whole microscope 37 °C chamber (custom designed by HMS Cell Biology machine shop), Semrock barrier filters (525/40, 607/36), Semrock dichroic mirror (405/488/568/647). Wavelengths of the excitation laser beam were 488 and 561 nm and fluorescence for mEGFP and mCherry was detected using 488/568 nm Yokogawa emission filter (Em01-R488/568-15, Semrock). Images were collected using the maximum field of view with 512 × 512 image size. Time-lapse images were collected with the frame acquisition rate ranged from 1.0 to 30 s per frame (indicated in the video legend). Immunofluorescence microscopy Cells were plated on a gelatin-coated chamber slide, transfected with PQ-FRET sensors, fixed with 4% formaldehyde in CB (10 mM MES pH 6.1, 138 mM KCl, 3 mM MgCl 2 , 2 mM EGTA) containing 0.32 M sucrose for 20 min, rinse in TBS (20 mM Tris–HCl pH7.4, 150 mM NaCl), permeabilized with 0.5% Triton X-100 in TBS for 10 min, rinse in TBS-0.1%Tx (TBS containing 0.1% Triton X-100), blocked in 2% BSA in TBS-0.1%Tx and incubated with Alexa568-phalloidin (Invitrogen, 1:200 dilution) or primary antibodies (mixture of mAb3-14 (5 μg ml −1 ) [16] and mAb1678 (5 μg ml −1 ), Millipore) for 1 h. After several washes with TBS-0.1%Tx, the cells were incubated with secondary antibodies (Invitrogen, 5 μg ml −1 ), washed with TBS-0.1%Tx, and mounted with mounting media (Spring Bioscience). Cells were imaged using a spinning-disk confocal microscope as described above with a 60 × /1.42 NA oil immersion objective (PLAPON 60XO, Olympus). FLNA-actin-myosin network To prepare nitrocellulose-coated slide glass and cover glass, the glasses were covered with 0.1% (v/v) collodion in amylacetate and air-dried. The surfaces were coated with human recombinant gelsolin (50 μg ml −1 ) in PBS for 1 min and blocked with 1% bovine serum albumin in blocking buffer (25 mM KCl, 20 mM Tris–HCl, 1 mM EGTA, 4 mM MgCl 2 , 10 mM DTT, pH 7.4) for 30 min. The coated surfaces were washed with the blocking buffer five times. Reconstituted networks were prepared by mixing 10 μM actin, 0.1 μM FLNA, 0.5 or 0.2 μM myosin (porcine cardiac myosin, Sigma M0531), 5 μM phalloidin and × 1 polymerization buffer (20 mM Tris_HCl, pH7.4, 50 mM NaCl, 0.5 mM EGTA, 4 mM MgCl 2 , 1 mM CaCl 2 , 5 mM DTT, 1 mM ATP; 1 mM γS-ATP was used for negative control) and sandwiched between the coated slide glass and cover glass with a 100 μm spacer (illustrated in Fig. 4 ). Each sample was allowed to polymerize for 1 h and fluorescence intensity was measured by spinning-disk confocal microscopy. Fluorescence intensities of mEGFP and mCherry were measured by NIH ImageJ and their ratio was calculated. Data analysis of PQ-FRET images Data sets were analysed using ImageJ 1.46j software (National Institutes of Health). A mEGFP/mCherry ratio image was created using ImageJ plugin ‘Ratio Plus’ and intensities of the ratio images were measured by ImageJ (Measure<Analyse or ‘Intensity v Time Monitor’<‘Stacks—T-functions’ plugins). The single steps for data processing are outlined in Supplementary Table 1 (ref. 60 ). Statistical analysis Excel and Prism were used to access statistical significance. How to cite this article: Nakamura, F. et al . Documentation and localization of force-mediated filamin A domain perturbations in moving cells. Nat. Commun. 5:4656 doi: 10.1038/ncomms5656 (2014).